Fibrinogen-induced perivascular microglial clustering is required for the development of axonal damage in neuroinflammation Blood-brain barrier disruption, microglial activation and neurodegeneration are hallmarks of multiple sclerosis. However, the initial triggers that activate innate immune responses and their role in axonal damage remain unknown. Here we show that the blood protein fibrinogen induces rapid microglial responses toward the vasculature and is required for axonal damage in neuroinflammation. Using in vivo two-photon microscopy, we demonstrate that microglia form perivascular clusters before myelin loss or paralysis onset and that, of the plasma proteins, fibrinogen specifically induces rapid and sustained microglial responses in vivo . Fibrinogen leakage correlates with areas of axonal damage and induces reactive oxygen species release in microglia. Blocking fibrin formation with anticoagulant treatment or genetically eliminating the fibrinogen binding motif recognized by the microglial integrin receptor CD11b/CD18 inhibits perivascular microglial clustering and axonal damage. Thus, early and progressive perivascular microglial clustering triggered by fibrinogen leakage upon blood-brain barrier disruption contributes to axonal damage in neuroinflammatory disease. Multiple sclerosis (MS) is a neuroinflammatory disease of unknown origin characterized by demyelination, axonal damage and disruption of the homeostatic balance between the vasculature and central nervous system (CNS) [1] . Recent histopathological analyses of pre-demyelinating MS lesions identified blood-brain barrier (BBB) disruption and activation of microglia, the resident immune cells in the CNS, as the earliest pathological signs in otherwise normal appearing white matter [2] , [3] . Microglial activation occurs in normal appearing white matter in the absence of lymphocyte infiltrates, suggesting that activation of innate immune responses might be critical for the development of autoimmunity [2] , [3] , [4] , [5] . Suppressing microglial activation in animal MS models reduces inflammatory demyelination and neurological deficits [6] , [7] . Moreover, in experimental autoimmune encephalomyelitis (EAE), an established animal model for MS, activation of microglia precedes infiltration of peripheral macrophages and occurs before disease onset [8] , [9] . Although ample evidence suggests that activation of microglia may represent one of the earliest events in neuroinflammatory disease, what triggers microglial activation in MS lesions, or precisely how and to what degree these early events relate to lesion formation and localized axonal damage remain unknown. Determining the signals that trigger activation of microglia in early disease stages is crucial for the development of therapies targeting MS pathogenesis. Microglia are critical in maintaining CNS homeostasis and form the first line of defense by regulating immunological and inflammatory responses [10] . However, it was not until microglia were studied in real time by in vivo two-photon laser scanning microscopy (2PLSM) that their dynamic behavior was appreciated in the healthy brain. Microglia perform tissue surveillance by continuously extending and retracting fine processes, while within only a few minutes after focal injury they extend processes to isolate damaged tissue [11] , [12] , [13] . In neurodegenerative pathologies such as Alzheimer’s disease, repetitive in vivo imaging showed microglial migration and association with newly forming plaques [14] . Although recent in vivo imaging studies have elegantly described the infiltration of T cells and their dynamic interaction with axons in EAE [15] , [16] , in vivo studies exploring in real time how microglia respond during neuroinflammation have not been performed. In vivo imaging with 2PLSM is a powerful tool to identify molecular triggers that induce rapid microglial responses and longitudinally study their behavior during the onset and progression of neuroinflammation. Here, we applied in vivo 2PLSM and recorded in real time the dynamic interactions between BBB disruption, microglia and axons during the course of EAE. We found a novel pattern of microglial motility toward the vasculature triggered by leakage of the plasma protein fibrinogen before onset of neurological signs, in the spinal cord of living mice undergoing EAE. We showed that fibrinogen induces release of reactive oxygen species (ROS) in microglia and its signaling through CD11b/CD18 is required for the formation of perivascular microglial clusters and axonal damage in EAE. These findings strongly support that fibrinogen-induced microglial clustering around the vasculature serves as a mechanism to facilitate lesion formation and focal axonal damage. Perivascular microglial clustering initiates before EAE onset To study the spatial and temporal regulation of microglial responses in neuroinflammatory disease, we performed time-lapse in vivo imaging in spinal cords of anesthetized Cx3cr1 GFP/+ mice after induction of EAE. In Cx3cr1 GFP/+ mice, enhanced green fluorescent protein (GFP) is expressed in resident CNS cells of the monocytic lineage [11] , [12] , [13] and, in particular, the CD45 low Ly6C low microglial population [17] . We used a spinal stabilization method we previously developed [12] and scanned the spinal cords from the leptomeninges up to ~250 μm deep in the parenchyma ( Supplementary Fig. S1 ). At the peak of disease, z -stack projections of the imaged volumes showed GFP-positive cells with thickened cell bodies and processes that formed high-density perivascular clusters ( Fig. 1a ). In control mice, cells were evenly distributed, stochastically extending and retracting their processes, contrary to increased cell density and activity within clusters at peak of disease ( Fig. 1a and Supplementary Movie 1 ). As early as 7 days post-immunization and before the onset of clinical EAE (clinical score: 0) ( Fig. 1b ), small-diameter clusters started to form in proximity to the vasculature ( Fig. 1a pre-onset). In pre-onset EAE, clusters were fewer in number than at peak of disease, but were still perivascular ( Fig. 1a ). Indeed, 98% of clusters imaged during EAE appeared in contact or within 30 μm of blood vessels ( Fig. 1d ). This proximity was independent of cluster size. In the chronic phase of EAE, the overall number of clusters was smaller than that at disease peak, and reduced progressively with time ( Fig. 1a-c ). The number of clusters correlates with clinical severity ( Fig. 1e , R 2 =0.7195; P <0.0001, F -test), suggesting that perivascular clusters are a strong pathological correlate of disease development. Further from the vasculature, increased cell body size of GFP + cells indicative of microglial activation was observed only at peak and chronic EAE, but not at pre-onset EAE ( Fig. 1f ). Overall, these results suggest that perivascular clustering is an early event in EAE pathogenesis that precedes parenchymal microglial activation. 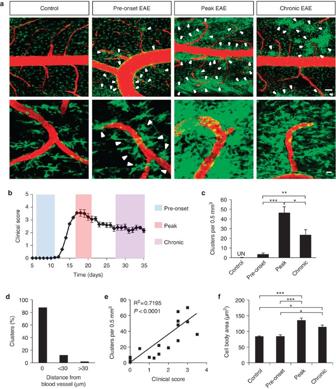Figure 1:In vivoimaging of perivascular microglial cluster formation at different stages of EAE. (a) Representative maximum projections ofz-stacks of images show microglia and pial macrophages (green) and the vasculature (red) in healthy (control), pre-symptomatic EAE (pre-onset EAE, clinical score 0), at the peak of clinical signs (peak EAE, mean clinical score 2.9), and at chronic EAE (mean clinical score 2.2). Arrowheads show areas of increased cell density appearing only in proximity to the vasculature. Images shown are from mice on days 8 (pre-onset), 17 (peak) and 31 (chronic) after induction of EAE. At least 10–15 mice were imaged per group. Scale bars, top: 100 μm; bottom: 20 μm. See correspondingSupplementary Movie 1. (b) EAE clinical score graph from a single representative experiment showing the timepoints selected for imaging during pre-onset, peak and chronic EAE. Values are mean±s.e.m.,n=10 mice. (c) Clusters were undetectable (UN) in healthy controls (n=5), but were detected in pre-onset EAE mice (n=5) and increased in number at peak (n=7) and chronic (n=5) EAE. Values are mean±s.e.m.*P<0.05, **P<0.01,***P<0.001 (one-way analysis of variance (ANOVA)). (d) 98% of clusters appeared in contact or within 30 μm from a blood vessel (data from 50 clusters in 12 mice). (e) Correlation analysis of the number of clusters with clinical score in EAE, at stages ranging from pre-onset to peak of disease. (n=22,R2=0.7195,P<0.0001,F-test). (f) Quantification of cell body size of non-clustered GFP+cells in control (n=5), pre-onset (n=6), peak (n=9), and chronic (n=4) EAE. On average 250 GFP+cells were measured per group. Values are mean±s.e.m., *P<0.05, ***P<0.001 (one-way ANOVA). Figure 1: In vivo imaging of perivascular microglial cluster formation at different stages of EAE. ( a ) Representative maximum projections of z -stacks of images show microglia and pial macrophages (green) and the vasculature (red) in healthy (control), pre-symptomatic EAE (pre-onset EAE, clinical score 0), at the peak of clinical signs (peak EAE, mean clinical score 2.9), and at chronic EAE (mean clinical score 2.2). Arrowheads show areas of increased cell density appearing only in proximity to the vasculature. Images shown are from mice on days 8 (pre-onset), 17 (peak) and 31 (chronic) after induction of EAE. At least 10–15 mice were imaged per group. Scale bars, top: 100 μm; bottom: 20 μm. See corresponding Supplementary Movie 1 . ( b ) EAE clinical score graph from a single representative experiment showing the timepoints selected for imaging during pre-onset, peak and chronic EAE. Values are mean±s.e.m., n =10 mice. ( c ) Clusters were undetectable (UN) in healthy controls ( n =5), but were detected in pre-onset EAE mice ( n =5) and increased in number at peak ( n =7) and chronic ( n =5) EAE. Values are mean±s.e.m. *P <0.05, * *P <0.01, ***P <0.001 (one-way analysis of variance (ANOVA)). ( d ) 98% of clusters appeared in contact or within 30 μm from a blood vessel (data from 50 clusters in 12 mice). ( e ) Correlation analysis of the number of clusters with clinical score in EAE, at stages ranging from pre-onset to peak of disease. ( n =22, R 2 =0.7195, P <0.0001, F- test). ( f ) Quantification of cell body size of non-clustered GFP + cells in control ( n =5), pre-onset ( n =6), peak ( n =9), and chronic ( n =4) EAE. On average 250 GFP + cells were measured per group. Values are mean±s.e.m., * P <0.05, *** P <0.001 (one-way ANOVA). Full size image Single-plane analysis at different depths ( Supplementary Fig. S2a ) and three-dimensional (3D) reconstruction of imaged volumes ( Fig. 2a and Supplementary Movie 2 ) showed perivascular clustering of pial macrophages and extensive clustering of microglia surrounding the branches of penetrating vessels in the spinal cord parenchyma. As determined by blood flow, most clusters that were imaged in vivo were localized around post-capillary venules and veins of the dorsal spinal cord. To further characterize the localization of the GFP + cells we performed immunostaining with an anti-pan laminin antibody, which detects the inner (endothelial) and outer (parenchymal) basement membranes [18] . GFP + cells were localized within the Virchow Robin space between the two basal laminae ( Supplementary Fig. S2b , arrows), and within the CNS parenchyma behind the glia limitans perivascularis ( Supplementary Fig. S2b , arrowheads), suggesting that in Cx3cr1 GFP/+ mice perivascular clusters consist of pial macrophages and microglia. In accordance with previous studies showing microglial proliferation in EAE [8] , [9] , GFP + cells proliferated within the clusters ( Supplementary Fig. S3 ), suggesting that increase in microglial and pial macrophage numbers in perivascular spaces is partly a result of local proliferation. 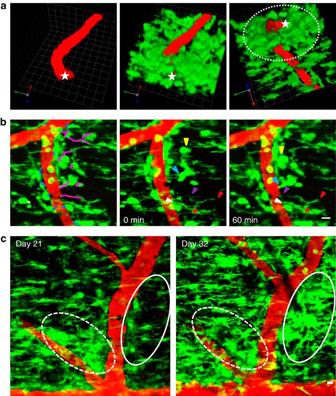Figure 2: Cluster formation and progression over the course of EAE. (a) 3D reconstruction of a representative spinal cord volume imagedin vivofrom the pial surface to 75 μm deep shows a pial vessel (red) in longitudinal orientation that turns perpendicularly and penetrates the spinal cord parenchyma (left). Overlay of the green channel shows the spatial relationship between GFP-positive cells and the vessel at the peak of EAE (middle). A full rotation showing the same volume of tissue from bottom to top shows increased accumulation of perivascular microglia around the parenchymal segment of the blood vessel (dotted line, right). The deepest point of the penetrating vessel is marked with white stars. Grid scale, 14 μm. See correspondingSupplementary Movie 2. (b) Time-lapsein vivoimaging showing pial macrophages and microglia rapidly associating with the vasculature at the peak of EAE. (Left) The leading edge of individual cell bodies or processes closest to the vasculature was tracked over a period of 60 min. Blue tracks identify cells that maintained their proximity to the vasculature and magenta tracks identify cells that either moved closer to the vasculature or extended processes toward it. (Middle and right) Yellow arrowheads show a cell approaching the blood vessel and associating with pre-existing perivascular cells over time. Blue arrowheads show a cell with processes already in contact with the blood vessel that migrates towards the vessel and eventually extends a new process toward it. Red star identifies a cell that maintains its point of contact with the vessel wall throughout the 60-min time course (white arrowheads), while it extends a new process toward the same blood vessel (magenta arrowheads), and retracts one of its processes that was directed away from the vessel (red arrowheads). Scale bar, 10 μm. See correspondingSupplementary Movie 3. (c) Repetitivein vivoimaging in the same spinal cord area 21 and 32 days after immunization shows a newly formed perivascular cluster (solid oval) on one side of a blood vessel and a resolving cluster (dotted oval) on the opposite side of the same vessel. Scale bar, 10 μm. Figure 2: Cluster formation and progression over the course of EAE. ( a ) 3D reconstruction of a representative spinal cord volume imaged in vivo from the pial surface to 75 μm deep shows a pial vessel (red) in longitudinal orientation that turns perpendicularly and penetrates the spinal cord parenchyma (left). Overlay of the green channel shows the spatial relationship between GFP-positive cells and the vessel at the peak of EAE (middle). A full rotation showing the same volume of tissue from bottom to top shows increased accumulation of perivascular microglia around the parenchymal segment of the blood vessel (dotted line, right). The deepest point of the penetrating vessel is marked with white stars. Grid scale, 14 μm. See corresponding Supplementary Movie 2 . ( b ) Time-lapse in vivo imaging showing pial macrophages and microglia rapidly associating with the vasculature at the peak of EAE. (Left) The leading edge of individual cell bodies or processes closest to the vasculature was tracked over a period of 60 min. Blue tracks identify cells that maintained their proximity to the vasculature and magenta tracks identify cells that either moved closer to the vasculature or extended processes toward it. (Middle and right) Yellow arrowheads show a cell approaching the blood vessel and associating with pre-existing perivascular cells over time. Blue arrowheads show a cell with processes already in contact with the blood vessel that migrates towards the vessel and eventually extends a new process toward it. Red star identifies a cell that maintains its point of contact with the vessel wall throughout the 60-min time course (white arrowheads), while it extends a new process toward the same blood vessel (magenta arrowheads), and retracts one of its processes that was directed away from the vessel (red arrowheads). Scale bar, 10 μm. See corresponding Supplementary Movie 3 . ( c ) Repetitive in vivo imaging in the same spinal cord area 21 and 32 days after immunization shows a newly formed perivascular cluster (solid oval) on one side of a blood vessel and a resolving cluster (dotted oval) on the opposite side of the same vessel. Scale bar, 10 μm. Full size image Continuous time-lapse imaging and cell tracking during cluster formation showed that perivascular cells exhibited multiple cell motility patterns. Cells in close proximity to the vasculature maintained their association with it, while cells further from the vasculature exhibited process extension and cell body movement directed toward the vasculature ( Fig. 2b and Supplementary Movie 3 ). Reimaging the same area of the spinal cord in the same mice on different days showed that while new perivascular clusters also formed at later disease stages, some pre-existing ones resolved ( Fig. 2c ). Thus, cluster formation around pial and parenchymal blood vessels begins before disease onset and continues throughout the course of neuroinflammatory disease. These findings reveal perivascular cluster formation as a novel pattern of microglial dynamics that occurs in parallel with pial macrophage accumulation toward the vasculature. Microglial clustering correlates with fibrin deposition As all the dynamic microglial responses were targeted toward the vasculature ( Figs 1 and 2 ), we hypothesized that a local vascular-derived signal might determine the direction of process extension and cell body movement. In human MS, BBB disruption occurs before the onset of inflammatory demyelination and precedes clinical symptoms [2] , [3] , [19] , [20] , [21] , [22] , [23] . To determine if BBB disruption is responsible for the early perivascular cluster formation, we performed real-time in vivo tracking of active BBB leakage in EAE. We observed rapid and progressive dye leakage from locally disrupted blood vessels that spatially correlated with the location of clusters, while cells at adjacent perivascular areas without dye leakage exhibited normal cell density ( Fig. 3a and Supplementary Movie 4 ). 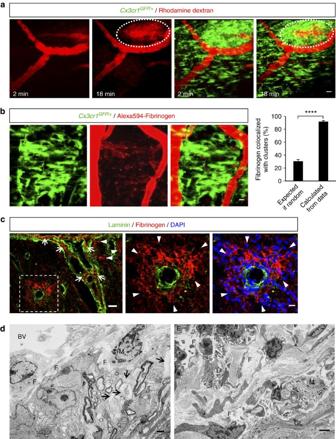Figure 3: Microglial clusters form in areas of BBB disruption and perivascular fibrin deposition. (a)In vivotime-lapse imaging in the spinal cord ofCx3cr1GFP/+EAE mice at the onset of clinical symptoms (clinical score 1) identified sites of active BBB disruption correlating with perivascular clusters. Imaging started immediately after a bolus i.v. injection of a 70 kDa rhodamine dextran solution (red). As time progressed, dye continuously leaked in the perivascular tissue that was occupied by an extensive microglial cluster (green). Scale bar, 20 μm. See correspondingSupplementary Movie 4. (b)In vivoimaging of microglial clusters (green) in the spinal cord ofCx3cr1GFP/+EAE-challenged mice after 3–7 daily i.v. injections of Alexa594-fibrinogen (red). Cluster formation overlaps with areas of perivascular fibrin deposition at the peak of EAE. The 91.8% calculated proportion of extracellular fibrin that colocalizes with microglia is significantly higher than the 30.6% predicted by Fisher’s combined probability test if the correlation were random. Bar graph represents mean±s.e.m. from 20 clusters fromn=8 mice injected with Alexa594-fibrinogen (****P<0.0001, pairedt-test). Scale bar, 10 μm. (c) Double immunofluorescence of laminin (basal membranes, green) and fibrin (red) shows fibrin deposition in the Virchow Robins space (arrows) as well as parenchymally (arrowheads, boxed area). Higher magnification images of the boxed area show parenchymal fibrin deposition correlating with perivascular inflammation shown with DAPI staining (blue). Scale bars, left: 30 μm; right: 10 μm. (d) Left: Correlated EM within the perivascular space of an inflamed spinal cord vessel shows abundant deposition of densely packed fibrillar material, consistent in ultrastructure with precipitated fibrin. The spinal cord parenchyma shows demyelinated fibers and dystrophic axons. Right: The perivascular space of a larger vessel contains abundant extracellular fibrillar material and macrophage/microglial cells with intracytoplasmatic lipid degradation products. (E, endothelial cell; F, fibrin; M, macrophage/microglia; GL, astrocytes of the glia limitans; BV, blood vessel; L, leukocyte, arrows: demyelinated/partly dystrophic axons). Scale bars, 2 μm. Figure 3: Microglial clusters form in areas of BBB disruption and perivascular fibrin deposition. ( a ) In vivo time-lapse imaging in the spinal cord of Cx3cr1 GFP/+ EAE mice at the onset of clinical symptoms (clinical score 1) identified sites of active BBB disruption correlating with perivascular clusters. Imaging started immediately after a bolus i.v. injection of a 70 kDa rhodamine dextran solution (red). As time progressed, dye continuously leaked in the perivascular tissue that was occupied by an extensive microglial cluster (green). Scale bar, 20 μm. See corresponding Supplementary Movie 4 . ( b ) In vivo imaging of microglial clusters (green) in the spinal cord of Cx3cr1 GFP/+ EAE-challenged mice after 3–7 daily i.v. injections of Alexa594-fibrinogen (red). Cluster formation overlaps with areas of perivascular fibrin deposition at the peak of EAE. The 91.8% calculated proportion of extracellular fibrin that colocalizes with microglia is significantly higher than the 30.6% predicted by Fisher’s combined probability test if the correlation were random. Bar graph represents mean±s.e.m. from 20 clusters from n =8 mice injected with Alexa594-fibrinogen ( ****P <0.0001, paired t- test). Scale bar, 10 μm. ( c ) Double immunofluorescence of laminin (basal membranes, green) and fibrin (red) shows fibrin deposition in the Virchow Robins space (arrows) as well as parenchymally (arrowheads, boxed area). Higher magnification images of the boxed area show parenchymal fibrin deposition correlating with perivascular inflammation shown with DAPI staining (blue). Scale bars, left: 30 μm; right: 10 μm. ( d ) Left: Correlated EM within the perivascular space of an inflamed spinal cord vessel shows abundant deposition of densely packed fibrillar material, consistent in ultrastructure with precipitated fibrin. The spinal cord parenchyma shows demyelinated fibers and dystrophic axons. Right: The perivascular space of a larger vessel contains abundant extracellular fibrillar material and macrophage/microglial cells with intracytoplasmatic lipid degradation products. (E, endothelial cell; F, fibrin; M, macrophage/microglia; GL, astrocytes of the glia limitans; BV, blood vessel; L, leukocyte, arrows: demyelinated/partly dystrophic axons). Scale bars, 2 μm. Full size image A prominent consequence of BBB leakage in MS is the local extravasation of plasma fibrinogen and other circulating hemostatic factors that results in the local deposition of perivascular fibrin matrices [21] . Fibrin deposition in active demyelinating MS lesions correlates with increased inflammatory activity [23] and microglial activation [24] . In early pre-demyelinating MS lesions, fibrin deposition and microglial activation are the first histopathological alterations, which precede the infiltration of T lymphocytes and demyelination [2] . Moreover, proteins traditionally associated with the control of hemostasis are highly expressed in MS brains [25] . To examine the role of fibrinogen in microglial clustering around the vasculature, we i.v. administered fluorescently labeled fibrinogen in Cx3cr1 GFP/+ mice daily, for 3–7 days during EAE. Quantification of in vivo imaging data revealed that 90% of the parenchymal fibrin deposition was associated with microglial clusters ( Fig. 3b ). Unlike dye, which gradually diffused in the CNS ( Fig. 3a ), fibrinogen leaked from the vasculature into the spinal cord parenchyma over a period of days and deposited as bright puncta, presumably due to its conversion to insoluble fibrin ( Fig. 3b ). In accordance with prior studies showing parenchymal fibrin deposition in EAE and MS [20] , [24] , [26] , [27] , immunohistochemical staining confirmed the presence of fibrin deposits both in the Virchow Robin space and in the CNS parenchyma, behind the glia limitans perivascularis ( Fig. 3c ). Moreover, correlated electron microscopy (EM) from previously imaged in vivo spinal cord regions ( Supplementary Fig. S1 ) further confirmed the presence of fibrillary extracellular deposits, consistent with polymerized fibrin fibrils, particularly around vessels in areas with demyelination and axonal damage ( Fig. 3d , left). Perivascular fibrillary deposits were closely attached to macrophage- or microglia-like cells with lysosomal inclusions, suggesting their phagocytic phenotype ( Fig. 3d , right). Thus, perivascular fibrin deposition may be a key spatial determinant of perivascular clustering in EAE. Fibrinogen induces rapid and sustained microglial responses To directly address whether fibrinogen was sufficient to trigger acute microglial responses in the CNS, we injected fibrinogen using a glass microelectrode into the cortex of Cx3cr1 GFP/+ mice and imaged microglial responses toward it in vivo . Injection of 5–10 pl of a 3–6 mg ml −1 fibrinogen solution (the physiological concentration of fibrinogen in plasma) caused rapid extension of microglial processes toward the tip of the electrode within ~30 min ( Fig. 4a and Supplementary Movie 5 ). Quantification showed a robust and statistically significant increase of microglial responses to fibrinogen compared with control injections of artificial cerebrospinal fluid (ACSF) or the blood protein albumin ( Fig. 4a ). Imaging of fibrin deposits over time showed that microglial clustering around fibrin was persistent and microglia remained closely associated with fibrin for at least 6 h ( Fig. 4b ). As neuroinflammatory disease occurs over the course of days to weeks, we examined whether fibrinogen-induced microglial activation also persisted for longer time periods. Indeed, fibrinogen induced microglial activation 3 days after stereotactic injection in the brain, in contrast to ACSF or albumin control ( Fig. 4c ). Like fibrinogen, wild-type plasma induced microglial activation three days after injection ( Fig. 4c ). In contrast, microglial activation was markedly lower after injection of Fib −/− plasma containing virtually every plasma protein with the exception of fibrinogen ( Fig. 4c ). Similarly, injection of plasma isolated from fibrinogen Fib γ390-396A knock-in mice, in which fibrinogen has been mutated to lack the CD11b/CD18 binding motif, yet it retains normal clotting function [28] , showed a reduction of microglial activation ( Fig. 4c ). Quantification showed significantly reduced microglial activation in response to Fib −/− or Fib γ390-396A plasma compared with wild-type plasma ( Fig. 4c ). Overall, these results suggest that upon increased vascular permeability in the CNS fibrinogen is sufficient and specific among plasma proteins to trigger microglial responses. 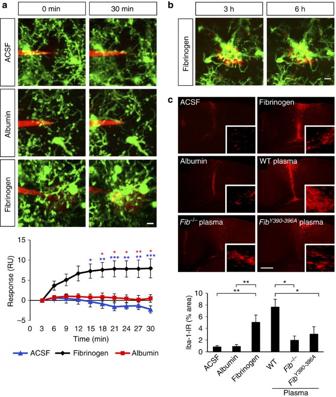Figure 4:Fibrinogen induces microglial responses in the healthy mouse cortexin vivo. (a) Local injection of fibrinogen (3–6 mg ml−1, red) in the cortex of theCx3cr1GFP/+mice causes microglial process extension (green) toward the tip of the injection electrode; control electrodes containing ACSF, or albumin (5 mg ml−1) caused little or no microglial responses. Quantification of microglial responses over 30 min toward the tip of the electrode upon injection of ACSF (n=7), albumin (n=6), or fibrinogen (n=9). (*P<0.05, **P<0.01, ***P<0.001, two-way analysis of variance (ANOVA)). Scale bar, 10 μm. See correspondingSupplementary Movie 5. (b) Sustained and prolonged microglial response in mouse cortex after a single injection of fibrinogen. Fibrinogen injected at a high concentration (6–10 mg ml−1, red) forms a deposit that is surrounded by microglial processes. The size of the fibrin deposit remains unaltered, and the microglial response to fibrin persists for at least 6 h. Scale bar, 10 μm. (c) Microglial immunoreactivity (Iba-1, red) and quantification from mouse brain sections 3 days after stereotactic injections of fibrinogen, ACSF or albumin protein control, or plasma isolated from wt,Fib−/−,Fibγ390-396Amice (n=6 mice per condition). Bar graph represents mean±s.e.m. (*P<0.05, **P<0.01, one-way ANOVA). Scale bar, 300 μm. Figure 4: Fibrinogen induces microglial responses in the healthy mouse cortex in vivo . ( a ) Local injection of fibrinogen (3–6 mg ml −1 , red) in the cortex of the Cx3cr1 GFP/+ mice causes microglial process extension (green) toward the tip of the injection electrode; control electrodes containing ACSF, or albumin (5 mg ml −1 ) caused little or no microglial responses. Quantification of microglial responses over 30 min toward the tip of the electrode upon injection of ACSF ( n =7), albumin ( n =6), or fibrinogen ( n =9). (* P <0.05, ** P <0.01, *** P <0.001, two-way analysis of variance (ANOVA)). Scale bar, 10 μm. See corresponding Supplementary Movie 5 . ( b ) Sustained and prolonged microglial response in mouse cortex after a single injection of fibrinogen. Fibrinogen injected at a high concentration (6–10 mg ml −1 , red) forms a deposit that is surrounded by microglial processes. The size of the fibrin deposit remains unaltered, and the microglial response to fibrin persists for at least 6 h. Scale bar, 10 μm. ( c ) Microglial immunoreactivity (Iba-1, red) and quantification from mouse brain sections 3 days after stereotactic injections of fibrinogen, ACSF or albumin protein control, or plasma isolated from wt, Fib −/− , Fib γ390-396A mice ( n =6 mice per condition). Bar graph represents mean±s.e.m. (* P <0.05, ** P <0.01, one-way ANOVA). Scale bar, 300 μm. Full size image Fibrin is required for perivascular microglial clustering Fibrinogen is not merely a marker of BBB disruption, but a major regulator of inflammatory demyelination [27] , [29] . To determine whether fibrinogen is necessary for cluster formation, we treated Cx3cr1 GFP/+ mice with anticoagulant during EAE and examined the formation of perivascular clusters in vivo . Increased fibrinolysis [30] or inhibition of fibrin formation with anticoagulants ameliorates clinical signs in EAE [25] , [27] , [29] . In vivo imaging showed that mice treated with the fibrin-depleting anticoagulant hirudin had a striking reduction in cluster formation ( Fig. 5a ). Moreover, correlated histopathological analysis of the same spinal cord segments previously imaged in vivo ( Supplementary Fig. S1 ) showed that hirudin also dramatically reduced fibrin deposition and demyelination ( Fig. 5b–d ). In contrast, untreated animals at the peak of EAE had extensive perivascular clustering shown by 2PLSM ( Fig. 5a ) associated with severe myelin loss with numerous phagocytic cells containing myelin degradation products ( Fig. 5c ), and extensive fibrin deposition ( Fig. 5b ). Importantly, clusters and fibrin deposition were present before the onset of EAE and preceded the appearance of demyelinating lesions ( Fig. 5a-d ). Moreover, there was a significant correlation between the number of clusters and fibrin deposition ( Fig. 5e , R 2 =0.5054; P <0.01, F- test) or the degree of demyelination ( Fig. 5e , R 2 =0.5692; P <0.001, F -test) in the same spinal cord volumes. In accordance to prior studies in EAE [15] and MS lesions [2] , infiltration of the CNS parenchyma by T cells was detected at the peak of disease ( Supplementary Fig. S4 ). Thus, fibrin is present in the CNS parenchyma before the onset of clinically apparent EAE and is necessary for perivascular cluster formation that precedes inflammatory demyelination. 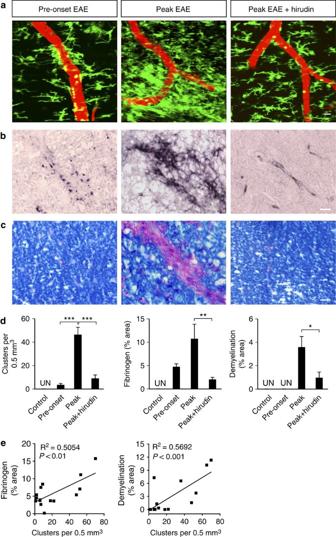Figure 5: Perivascular cluster formation requires fibrin deposition and precedes demyelination. Representativein vivoimages (a) and correlated histology (b,c) from the same mice are shown at pre-onset EAE, peak EAE, and peak EAE after hirudin administration. (a)In vivoimaging of microglial clusters (green) in relation to the vasculature (red) in the mouse EAE spinal cord. Scale bar, 10 μm. (b) Fibrinogen immunoreactivity. Scale bar, 10 μm. (c) Myelin staining with LFB (blue) counterstained with PAS (phagocytes, purple). Scale bar, 10 μm. (d) Number of clusters, fibrinogen immunoreactivity and demyelination in the spinal cord of healthy, EAE, and hirudin-treated mice. In healthy controls (n=5), microglial clusters, fibrin and demyelination were undetectable (UN). In pre-onset EAE (n=5), microglial clusters and fibrin were present, but there was no demyelination. At the peak of EAE, there was an increase in microglial clusters (n=9), fibrin deposition (n=7) and demyelination (n=8). At the peak of EAE in hirudin-treated mice (n=9), microglial clusters, fibrin deposition and demyelination were significantly reduced. Values are mean±s.e.m.**P<0.01,***P<0.001 (one-way analysis of variance (ANOVA)),*P<0.05 (Mann–Whitney test). (e) Correlation analysis of the number of clusters with fibrin deposition (n= 15,R2=0.5054,P<0.01,F-test) and demyelination (n=16,R2=0.5692,P<0.001,F-test). Figure 5: Perivascular cluster formation requires fibrin deposition and precedes demyelination. Representative in vivo images ( a ) and correlated histology ( b,c ) from the same mice are shown at pre-onset EAE, peak EAE, and peak EAE after hirudin administration. ( a ) In vivo imaging of microglial clusters (green) in relation to the vasculature (red) in the mouse EAE spinal cord. Scale bar, 10 μm. ( b ) Fibrinogen immunoreactivity. Scale bar, 10 μm. ( c ) Myelin staining with LFB (blue) counterstained with PAS (phagocytes, purple). Scale bar, 10 μm. ( d ) Number of clusters, fibrinogen immunoreactivity and demyelination in the spinal cord of healthy, EAE, and hirudin-treated mice. In healthy controls ( n= 5), microglial clusters, fibrin and demyelination were undetectable (UN). In pre-onset EAE ( n= 5), microglial clusters and fibrin were present, but there was no demyelination. At the peak of EAE, there was an increase in microglial clusters ( n =9), fibrin deposition ( n= 7) and demyelination ( n= 8). At the peak of EAE in hirudin-treated mice ( n =9), microglial clusters, fibrin deposition and demyelination were significantly reduced. Values are mean±s.e.m. **P <0.01, ***P <0.001 (one-way analysis of variance (ANOVA)), *P <0.05 (Mann–Whitney test). ( e ) Correlation analysis of the number of clusters with fibrin deposition ( n = 15, R 2 =0.5054, P <0.01, F- test) and demyelination ( n =16, R 2 =0.5692, P <0.001, F- test). Full size image Axonal damage in neuroinflammation requires fibrinogen As innate immune responses contribute to axonal damage [2] , [31] , [32] , [33] , we examined the role of fibrinogen-induced perivascular microglial clusters in lesion formation in EAE. We performed simultaneous three-color in vivo imaging of i.v. injected fluorescent fibrinogen in Cx3cr1 GFP/+ / Thy1-CFP mice, in which microglia are labeled with GFP and axons with cyan fluorescent protein (CFP) [34] . In healthy mice, axons near blood vessels were structurally intact ( Fig. 6a , control). However, mice at peak EAE had evident signs of axonal deformities, such as blebbing, bending and fragmentation, in the vicinity of fibrin deposits and perivascular clusters ( Fig. 6a , peak EAE). Fibrin deposition correlates with axonal damage in early [2] and active [35] MS lesions. To determine if fibrin is required for axonal damage in neuroinflammation, we performed anticoagulant treatment in Cx3cr1 GFP/+ / Thy1-CFP mice, followed by in vivo imaging and a correlated histopathological analysis of the same spinal cord area with SMI-32, a marker for non-phosphorylated neurofilament that indicates axonal damage. In healthy controls, evenly distributed microglia exhibited baseline extension/retraction motility of their finer processes between intact axons ( Fig. 6b and Supplementary Movie 6 , control), which showed no signs of degeneration by SMI-32 staining ( Fig. 6b , control). At the peak of EAE, clustered microglia wrapped around axons characterized by evident signs of damage (bending, swelling, fragmentation) ( Fig. 6b , peak EAE) and demonstrated increased SMI-32 staining indicative of axonal degeneration ( Fig. 6b , peak EAE). Time-lapse in vivo imaging showed axons undergoing abrupt morphological distortions that correlated with the relative motion of proximal microglial cell bodies or processes within the clusters ( Supplementary Movie 6 , peak EAE). Living axonal segments still expressing CFP appeared to be detached by neighboring microglial processes within minutes ( Supplementary Movie 7 ). In accordance with engulfment of axonal debris by microglia in MS lesions [36] , high resolution confocal microscopy showed SMI-32 labeled axonal fragments engulfed by microglia ( Fig. 6c ). The total number of clusters significantly correlated with axonal damage in the EAE spinal cord ( Fig. 6d ; R 2 =0.8804, P <0.0001, F -test). Strikingly, upon anticoagulant treatment microglial distribution and interactions with axons in EAE were similar to healthy control ( Fig. 6b and Supplementary Movie 6 , peak EAE+hirudin), and SMI-32 immunoreactivity was dramatically reduced ( Fig. 6b , peak EAE+hirudin). 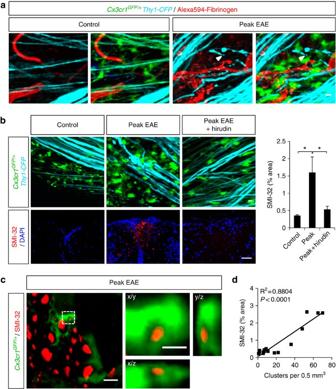Figure 6: Fibrinogen is required for development of axonal damage in neuroinflammation. (a) Simultaneousin vivoimaging of GFP-expressing microglia (green), CFP-expressing axons (cyan) and Alexa594-fibrinogen-injected blood vessels (red) in the EAE spinal cord. Axonal damage in the form of blebbing, bending, constrictions and fragmentation (arrowheads) is evident mostly near perivascular microglial clusters, in areas with fibrin deposits. Scale bar, 10 μm. (b)In vivoimaging shows reduced microglial clustering and axonal deformities after anticoagulant treatment. In healthy control (n=5), microglia show even distribution between structurally intact axons. At the peak of EAE (n=9), there are extensive signs of axonal structural abnormalities within areas of microglial clusters. At the peak of EAE, the anticoagulant hirudin (n=12) significantly reduces microglial clustering and morphologic signs of axonal damage. See correspondingSupplementary Movies 8 and 9. Correlated histology using SMI-32, a marker of axonal damage, performed in the same spinal cord area imagedin vivo, shows a decrease of SMI-32-labelled axons in the hirudin-treated mice (n=11), compared with untreated mice at the peak of EAE (n=8). Values are mean±s.e.m.*P<0.05 (one-way analysis of variance (ANOVA)). Scale bars, top: 10 μm; bottom: 50 μm. (c) High resolution confocal microscopy of SMI-32 stained spinal cord sections shows engulfment of axonal fragments (red) by microglia (green). Boxed area is shown in x/y, x/z and y/z projections to confirm the intracellular localization of an axonal fragment within a microglial cell body. Scale bars, left: 10 μm; right: 2 μm. (d) Correlation analysis of the number of clusters with axonal damage (n=16,R2=0.8804,P<0.0001,F-test). Figure 6: Fibrinogen is required for development of axonal damage in neuroinflammation. ( a ) Simultaneous in vivo imaging of GFP-expressing microglia (green), CFP-expressing axons (cyan) and Alexa594-fibrinogen-injected blood vessels (red) in the EAE spinal cord. Axonal damage in the form of blebbing, bending, constrictions and fragmentation (arrowheads) is evident mostly near perivascular microglial clusters, in areas with fibrin deposits. Scale bar, 10 μm. ( b ) In vivo imaging shows reduced microglial clustering and axonal deformities after anticoagulant treatment. In healthy control ( n= 5), microglia show even distribution between structurally intact axons. At the peak of EAE ( n= 9), there are extensive signs of axonal structural abnormalities within areas of microglial clusters. At the peak of EAE, the anticoagulant hirudin ( n= 12) significantly reduces microglial clustering and morphologic signs of axonal damage. See corresponding Supplementary Movies 8 and 9 . Correlated histology using SMI-32, a marker of axonal damage, performed in the same spinal cord area imaged in vivo , shows a decrease of SMI-32-labelled axons in the hirudin-treated mice ( n= 11), compared with untreated mice at the peak of EAE ( n= 8). Values are mean±s.e.m. *P <0.05 (one-way analysis of variance (ANOVA)). Scale bars, top: 10 μm; bottom: 50 μm. ( c ) High resolution confocal microscopy of SMI-32 stained spinal cord sections shows engulfment of axonal fragments (red) by microglia (green). Boxed area is shown in x/y, x/z and y/z projections to confirm the intracellular localization of an axonal fragment within a microglial cell body. Scale bars, left: 10 μm; right: 2 μm. ( d ) Correlation analysis of the number of clusters with axonal damage ( n =16, R 2 =0.8804, P <0.0001, F- test). Full size image Reactive oxygen and nitric oxide intermediates are produced through the induction of the respiratory burst in activated microglia and are major candidates for the induction of axon degeneration in inflammatory demyelination [37] , [38] , [39] . At the peak of EAE, in vivo ROS generation specifically increased within microglial clusters compared with normal density areas or healthy controls ( Fig. 7a ). In vitro , treating microglia with fibrinogen, induced a 5.1-fold increase of H 2 O 2 and a 7.4-fold increase in iNOS gene expression ( Fig. 7b ). Overall, these findings suggest that fibrinogen might contribute to the ROS generation in inflammatory demyelinating lesions and show that perivascular fibrin deposition is required for axonal degeneration within microglial clusters in neuroinflammatory disease. 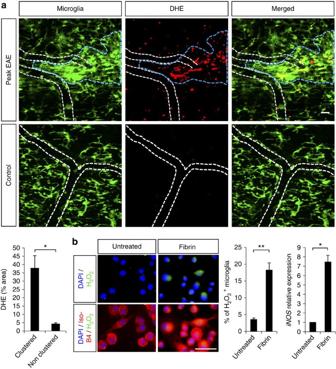Figure 7: Fibrin induces ROS generation in microglia. (a)In vivoimaging of microglial clusters (green) in the spinal cord ofCx3cr1GFP/+EAE-challenged mice after 2 daily i.v. injections of the superoxide indicator dihydroethidium (DHE, red). A significant increase of DHE signal was detected within clustered areas (blue dotted line) compared with neighboring non-clustered areas in the same animals at the peak of EAE, as well as to healthy controls. White dotted lines outline blood vessels. Bar graph represents mean±s.e.m. fromn=4 mice (*P<0.05, Mann–Whitney test). Scale bar, 20 μm. (b) H2O2production shown by the PYME probe (green) in BV2 microglia labeled with IsoB4 (red) after treatment with fibrinD-dimer. Quantification of cells positive for H2O2expressed as a percentage of total cell number. Values are mean±s.e.m. from untreated,n=6 wells, 1481 cells counted; fibrin D-dimer,n=7 wells, 1172 cells counted,**P<0.01 (Mann–Whitney test). Real-time PCR ofiNOSgene expression in BV2 cell extracts upon fibrinogen treatment.n=2 independent experiments performed in triplicates,*P<0.05 (Mann–Whitney test). Scale bar, 50 μm. Figure 7: Fibrin induces ROS generation in microglia. ( a ) In vivo imaging of microglial clusters (green) in the spinal cord of Cx3cr1 GFP/+ EAE-challenged mice after 2 daily i.v. injections of the superoxide indicator dihydroethidium (DHE, red). A significant increase of DHE signal was detected within clustered areas (blue dotted line) compared with neighboring non-clustered areas in the same animals at the peak of EAE, as well as to healthy controls. White dotted lines outline blood vessels. Bar graph represents mean±s.e.m. from n =4 mice ( *P <0.05, Mann–Whitney test). Scale bar, 20 μm. ( b ) H 2 O 2 production shown by the PYME probe (green) in BV2 microglia labeled with IsoB4 (red) after treatment with fibrin D -dimer. Quantification of cells positive for H 2 O 2 expressed as a percentage of total cell number. Values are mean±s.e.m. from untreated, n =6 wells, 1481 cells counted; fibrin D-dimer, n =7 wells, 1172 cells counted, **P <0.01 (Mann–Whitney test). Real-time PCR of iNOS gene expression in BV2 cell extracts upon fibrinogen treatment. n =2 independent experiments performed in triplicates, *P <0.05 (Mann–Whitney test). Scale bar, 50 μm. Full size image Axonal damage requires fibrin signaling via CD11b/CD18 Fibrinogen is a ligand for the microglial integrin receptor CD11b/CD18, and this interaction regulates the development of clinical disease in EAE [27] . To examine the contribution of the CD11b/CD18 receptor to fibrinogen-mediated microglial cluster formation and axonal damage, we crossed Cx3cr1 GFP/+ mice with Fib γ390-396A mice. Fib γ390-396A mice show normal clotting function and fibrin deposition in vivo and no differences in circulating leukocyte numbers or trafficking [27] , [28] . In vivo imaging of the gliovascular interface in EAE-challenged Cx3cr1 GFP/+ Fib γ390-396A mice revealed significant reduction of microglial clustering ( Fig. 8a ). Moreover, correlated histopathological analysis showed that axons were also significantly protected from degeneration in Cx3cr1 GFP/+ Fib γ390-396A mice ( Fig. 8a , SMI-32). These findings suggest that fibrinogen signaling through CD11b/CD18 regulates perivascular microglial responses in the CNS and contributes to axonal damage and localized lesion formation in neuroinflammatory disease. 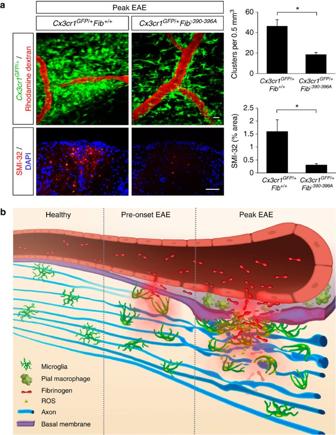Figure 8: Fibrinogen mediates perivascular microglial clustering and axonal damage via CD11b/CD18. (a)In vivoimaging ofCx3cr1GFP/+Fibγ390-396Amice at the peak of EAE (n=6) shows fewer perivascular clusters (top) and significantly less SMI-32 immunoreactivity (bottom) than inCx3cr1GFP/+Fib+/+controls (n=9). Correlated histology was performed in the same spinal cord areas in the mice that were previously imagedin vivo. Values are mean±s.e.m.*P<0.05 (Mann–Whitney test). Scale bars, top: 10 μm; bottom: 50 μm. (b) Schematic illustration and working model of the dynamic responses of perivascular microglia and pial macrophages to BBB disruption and their contribution to axonal damage in neuroinflammatory disease. In the healthy CNS, microglia are evenly distributed and stochastically extend and retract their processes. In EAE mice before the onset of neurological symptoms fibrinogen leaks in the CNS, triggering microglial process extension and cell body accumulation toward the vasculature. At the peak of disease, microglial clustering around the vasculature occurs almost exclusively in areas of fibrin deposition and is associated with axonal damage and release of ROS by microglia. Fibrinogen signaling via the CD11b/CD18 integrin receptor is required for the formation of perivascular clusters and the development of axonal damage. Figure 8: Fibrinogen mediates perivascular microglial clustering and axonal damage via CD11b/CD18. ( a ) In vivo imaging of Cx3cr1 GFP/+ Fib γ390-396A mice at the peak of EAE ( n =6) shows fewer perivascular clusters (top) and significantly less SMI-32 immunoreactivity (bottom) than in Cx3cr1 GFP/+ Fib +/+ controls ( n= 9). Correlated histology was performed in the same spinal cord areas in the mice that were previously imaged in vivo . Values are mean±s.e.m. *P <0.05 (Mann–Whitney test). Scale bars, top: 10 μm; bottom: 50 μm. ( b ) Schematic illustration and working model of the dynamic responses of perivascular microglia and pial macrophages to BBB disruption and their contribution to axonal damage in neuroinflammatory disease. In the healthy CNS, microglia are evenly distributed and stochastically extend and retract their processes. In EAE mice before the onset of neurological symptoms fibrinogen leaks in the CNS, triggering microglial process extension and cell body accumulation toward the vasculature. At the peak of disease, microglial clustering around the vasculature occurs almost exclusively in areas of fibrin deposition and is associated with axonal damage and release of ROS by microglia. Fibrinogen signaling via the CD11b/CD18 integrin receptor is required for the formation of perivascular clusters and the development of axonal damage. Full size image By in vivo imaging of BBB disruption, microglia and axons, we identified fibrinogen as a novel molecular signal that triggers rapid perivascular microglial responses, and contributes to axonal damage in neuroinflammatory disease. Intriguingly, microglia exhibit cell motility patterns directed specifically toward the vasculature that precede the onset of neurological signs and lesion formation. Therefore, our data suggest that BBB disruption is necessary for the mobilization of the resident innate immune cells around the CNS vasculature, which might represent one of the earliest events in MS pathology that can trigger and amplify inflammatory demyelination and axonal damage ( Fig. 8b ). Our study demonstrates a novel pattern of microglial motility toward the vasculature not previously observed in other injury or disease models. In contrast to Alzheimer’s disease [14] and laser-induced injury [11] , [13] , in neuroinflammation, microglia primarily respond to the vasculature by a combination of process extension and cell body motility. Microglial responses toward the vasculature occur already at the pre-onset stage of EAE. As demyelination and axonal damage are prominent at the peak of EAE as shown in our study and previously [31] , microglial clusters might demarcate the areas of new lesion formation. Extensive axonal deformities appear in synchrony with rapid microglial process extension and retraction, and such events were recorded only perivascularly, at sites of BBB leakage with fibrin deposition and not in other areas in the parenchyma. Although this might be a real-time in vivo representation of the classic role of microglia as phagocytic cells that remove cellular debris, microglia might have a primary role in axonal destruction. Indeed, as we recorded multiple microglial interactions with abnormal axonal formations and fragments still expressing CFP, and confirmed with confocal microscopy engulfment of axonal fragments by microglia, we postulate that microglia might attack and phagocytose living axonal fragments at areas of BBB leakage. This agrees with the observations that microglia and macrophages are close to degenerating axons with intact myelin sheaths [40] , and phagocytosis of axonal fragments by microglia occurs in MS lesions [36] . Therefore, our three-color in vivo imaging studies identify the vasculature as a niche for activation of innate immune responses and axonal damage in neuroinflammation. Furthermore, they support neuropathological studies in MS plaques that have suggested a primary role for microglia and their inflammatory activity in axonal damage [41] , [42] , [43] . Our study reveals a novel function for fibrinogen as a signal that induces rapid, yet sustained microglial responses in vivo in the healthy brain. In vivo real-time imaging previously identified rapid microglial process extension upon injection of ATP [11] . Fibrinogen is a novel molecular signal that can mediate a similar response. ATP mediates microglial responses through the P 2 Y 12 receptor [44] . As rapid microglial process extension is associated with dramatic cytoskeletal rearrangements, presumably involving activation of the Rho signaling pathway, cross-talk of P 2 Y 12 with integrin receptors might mediate the rapid microglial response induced by fibrinogen. Indeed, integrins are primarily responsible for cytoskeletal rearrangements, and fibrinogen induces Rho activation in microglia via CD11b/CD18 (ref. 27 ). ATP induces integrin-β1 expression in microglia through P 2 Y 12 receptor and integrin-β1 activation is involved in the directional process extension by microglia in brain tissue [45] . Moreover, ATP increases CD11b expression in microglia [46] and eosinophils [47] . Future studies will determine the potential cross-talk between P 2 Y 12 and microglial integrin receptors upon BBB disruption. The perivascular responses we observe are not restricted to microglia, but also include the resident pial macrophages. Meningeal and parenchymal blood vessels have different architecture, as leptomeningeal blood vessels are not surrounded by the glia limitans perivascularis. Interestingly, we observe fibrin deposition and perivascular clustering around both meningeal and parenchymal blood vessels. The concomitant responses of microglia and resident pial macrophages to BBB leakage imply an aspect of functional convergence of the two CNS-resident monocytic populations in perivascular clustering during neuroinflammatory disease. Fibrin/CD11b signaling appears to mediate both responses of microglia and pial macrophages, since anticoagulant treatment or studies in the Fib γ390-396A mice ameliorate responses of both cell populations (our study) and clinical EAE severity [25] , [27] . Although our study demonstrated the interplay between BBB disruption with the Cx3cr1 GFP/+ CNS-resident microglia and pial macrophages, fibrin/CD11b signaling might also be responsible for peripheral macrophage recruitment in neuroinflammation. Infiltration of peripheral monocytes in the CNS parenchyma is crucial for disease progression and depends on CCR2 expression [8] , [17] . Cx3cr1 GFP/+ mice are primarily reporters for resident monocytes [17] . In the Cx3cr1 GFP/+ mice there are only a few peripherally circulating GFP-positive cells, which are not expressing CCR2 [17] , suggesting that these cells do not infiltrate in the CNS. Future studies with differentially labeled resident and peripheral monocyte populations will dissect the role of fibrinogen in macrophage recruitment in CNS disease. Thus, molecular events at the BBB that trigger early perivascular plasma leakage and immune cell clustering may regulate peripheral inflammatory responses and infiltration of the CNS. A fundamental question in the development of inflammatory demyelination has been the identity of the early triggers and the amplifiers of disease pathogenesis. It is considered axiomatic that large-scale transmigration across the BBB is associated with loss of barrier function. Studies from neuropathology in early MS lesions that showed fibrin deposition and microglial activation in the absence of parenchymal T cells or demyelination suggested that there are other mechanisms in play that might open the BBB and activate microglia [2] , [3] , [4] , [5] . However, standard histopathology techniques cannot decipher which comes first (that is, microglial activation or BBB disruption). Our study shows that fibrinogen that enters into the CNS after BBB leakage is sufficient and specific among blood proteins to trigger rapid microglial responses even in the healthy CNS in the absence of a pre-existing lesion. Thus, it is possible that in genetically susceptible individuals, early events at the gliovascular interface, such as fibrinogen leakage in the CNS, might function as triggers that are sufficient to promote autoimmune responses resulting in further BBB disruption, demyelination and plaque formation. Indeed, CD11b-positive monocytes modulate autoimmune responses [48] and perivascular microglia and pial macrophages have properties of antigen-presenting cells [49] , [50] , [51] . Therefore, early cluster formation mediated by fibrin/CD11b signaling may contribute to the development of autoimmunity. These mechanisms might also be in play in active MS plaques, where release of proinflammatory cytokines by infiltrating macrophages and T cells may further open the BBB and enhance fibrin deposition in the CNS. Similar to microglia, astrocyte activation also occurs early in EAE before significant T-cell entry, and is associated with axonal damage in the optic nerve [52] . As fibrinogen induces astrocyte activation [53] , it is possible that it might also contribute to the early activation of astrocytes in neuroinflammation. Identifying fibrinogen as a trigger for perivascular microglial activation in early disease stages is crucial for the understanding of microglial functions and their contribution to CNS autoimmune disease as well as for the development of therapies targeting early stages in MS pathogenesis. Future in vivo imaging studies using differentially labeled lymphocytes, peripheral macrophages, microglia, astrocytes and fibrinogen will establish the temporal and spatial relationships that govern adaptive and innate immune responses during the course of EAE. Microglia and macrophages are considered main effector cells of the innate immune response in the CNS that might be involved in axonal damage [32] . In MS lesions, a major mechanism of axonal damage is related to the effects of ROS, which may lead to axonal damage via mitochondrial impairment [54] . In accordance, neutralization of ROS in EAE reduced axonal damage [40] . We show that fibrinogen induces ROS release in microglia and that its signaling via the microglial receptor CD11b is required for development of axonal damage in inflammatory disease. Fibrin deposition correlates with acute axonal damage and microglial activation in early pre-demyelinating MS lesions before the infiltration of lymphocytes [2] . Moreover, fibrin accumulates on demyelinated axons in chronic-progressive MS [21] , [35] . Axonal damage is considered a critical cause of disability in MS and is associated with activation of the innate immune system, suggesting that suppressing innate immune responses could be an important therapeutic strategy for progressive MS [42] . Therefore, targeting the interactions of fibrinogen with the CD11b/CD18 integrin receptor might be a potent new therapeutic approach to suppress the activation of innate immune responses and prevent axonal damage in neuroinflammatory disease. Animals Cx3cr1 GFP/+ (ref. 55 ) and Thy1-CFP (ref. 34 ) mice were obtained from Jackson Laboratory. Fib −/− (ref. 56 ) and Fib γ390-396Α mice [28] were also used. Cx3cr1 GFP/+ mice were crossed to Fib γ390-396Α and Thy1-CFP mice to generate Cx3cr1 GFP/+ Fib γ390-396Α and Cx3cr1 GFP/+ Thy1-CFP mice. All mice used were female and on C57Bl/6 background. EAE using MOG 35-55 was induced as described [27] . Blood vessels were labeled by intravenous (i.v.) injections of 3% rhodamine dextran (70 kDa or 2 MDa) (Invitrogen). Alexa594-Fibrinogen (Invitrogen) was administered daily for 3–7 days (5 mg kg −1 , i.v.) and during imaging. All animal procedures were performed under the guidelines set by Institutional Animal Care and Use Committees at the University of California, San Diego and the University of California, San Francisco. In vivo multiphoton microscopy We used a Radiance-2000 multiphoton microscope (Bio-Rad) with a Millenia/Tsunami laser (Spectra Physics), Fluoview FV1000MPE (Olympus) and an Ultima-IV multiphoton microscope (Prairie) both equipped with MaiTai DeepSee-eHP lasers (Spectra Physics). The excitation wavelength was tuned to 880–915 nm. Imaging was performed from the surface to ~250 μm below the pia, using an Olympus 40 × 0.8 NA, or a Nikon a 40 × 0.8 NA or a Nikon 10 × 0.4 NA water-immersion lenses with either a 1.0–1.5-μm or a 3–4-μm z -step, for 40 × or 10 × magnification respectively. For time-lapse imaging, a z -stack of images was acquired every 120–240 s, typically over 30–90 min. In vivo imaging in the mouse spinal cord In vivo spinal cord imaging was performed as described [12] . Briefly, the spinal cord was exposed through a single laminectomy, and mice were positioned on a spinal stabilization device. This technique allows imaging of microglial dynamics without inducing perturbation of the pial vessels or inflammatory responses in the spinal cord [12] . We confirmed in control mice the absence of surface injury related to this procedure over a 2-h observation period (not shown); animals that sustained accidental injury during the laminectomy were excluded from the study. For reimaging the same spinal cord areas on different days, in vivo imaging was performed between adjacent vertebral arches, leaving bone structures intact, but after carefully removing interlaminar tissue to avoid microglial activation in the underlying spinal cord [57] . The vasculature was used as a map to relocate previously imaged areas, and reimage them in vivo [12] . At the end of each imaging session, back muscles and skin were restored and sutured, and animals were given appropriate postoperative care [12] . In vivo imaging and injections in the mouse brain In vivo imaging in the cortex was performed as described [11] . Glass electrodes loaded with 3–10 mg ml −1 Alexa594-fibrinogen, or 3% rhodamine dextran, or 5 mg ml −1 Alexa594-Albumin (Invitrogen) all diluted in ACSF were inserted 50 μm into the cortex with a micromanipulator (Narishige), using epifluorescence guidance. A small volume (~5–10 pl) was injected in the cortex with a pressure injector (Eppendorf), while cell responses were monitored by in vivo imaging. Processing of in vivo imaging data Z -stacks of images were projected along the z -axis to recreate two-dimensional representations of the 3D structures within the imaged volumes. 3D reconstruction and volume rendering was performed using Volocity (PerkinElmer). Time-lapse movies were generated using z projections of stacks acquired sequentially over time, and were in some cases aligned. Images and movies were adjusted for brightness, contrast and background noise with ImageJ (NIH). To separate the overlapping signals from CFP-expressing axons and GFP-expressing microglia, the detection scheme was optimized by selecting narrow, non-overlapping bandpass filters and a 495-nm dichroic mirror (Chroma). The spectral unmixing algorithm in ImageJ was used to separate the two signals, which were subsequently pseudocolored. Cell tracking was performed with the TrackJ algorithm. Quantification of cell clusters and sizes Z -stacks of images from Cx3cr1 GFP/+ healthy control or EAE-challenged mice were z -projected and automatically thresholded (maximum entropy algorithm of ImageJ), to account for signal intensity differences between experiments. Cell density differences were computed by calculating the percent of white (255-value) pixels in same-size regions of interest drawn in each z -projection. Cluster number, diameter and distance to the closest blood vessel were measured with ImageJ. Clusters were defined as areas where cell density was at least two-fold higher than in healthy appearing spinal cord. Cell body area was measured in non-thresholded projections also with ImageJ. Proliferation assay Mice were injected i.p. with 50 mg kg −1 5-ethynyl-2′-deoxyuridine (EdU) for two consecutive days. 24 h after last EdU injection mice were transcardially perfused with 4% paraformaldehyde (PFA) in PBS, spinal columns were excised and postfixed in PFA for 12 h. EdU was labelled in spinal cord explants using the Alexa647 Click-iT EdU Imaging kit (Molecular Probes). Imaging of the dorsal side of spinal cord explants was performed with an Olympus Fluoview 1000 confocal microscope using an Olympus 20 × 1.05 NA water-immersion lens. Colocalization analysis of extravasated fibrinogen and cell clusters z -stacks of images were acquired in green and red channels simultaneously and subsequently z -projected. The extravascular red signal (corresponding to Alexa594-fibrinogen) and the green channel (corresponding to cells) were automatically thresholded as described above. The resulting image for each channel was converted to a text image, a tabular format where a value of 0 (no fluorescence) or 255 (fluorescence) was assigned for each pixel. A binomial test implemented in R (R Foundation), was used to compare corresponding pixel values in the two channels. We calculated colocalization of red and green fluorescence in corresponding pixels compared with random association. Anticoagulation Four days after immunization, mice were injected daily with lepirudin (recombinant hirudin; Refludan, Bayer), 10 mg kg −1 i.p. in 0.9% NaCl solution [25] . Controls received an equal volume (100 μl) of 0.9% NaCl. Plasma isolation Blood was collected from the inferior vena cava of anesthetized mice into one-tenth volume of 0.129 M sodium citrate (Becton Dickinson) as described [28] , [56] . Plasma was prepared by centrifugation at 2,500 g for 10 min at room temperature. Stereotactic injections Mice were anesthetized with avertin and placed in a stereotaxic apparatus (Kopf Instruments). Fibrinogen (Calbiochem) was dissolved in endotoxin-free distilled water (HyClone), diluted to 5 mg ml −1 with ACSF. 1 μl of 5 mg ml −1 fibrinogen, ACSF, or 5 mg ml −1 albumin or 3 μl of plasma solutions were slowly injected (0.3 μl min −1 ) with a 10-μl Hamilton syringe and a 33-gauge needle stereotactically inserted into the corpus callosum of C57Bl/6 mice as described [53] . Correlated histology and light microscopy After in vivo imaging, mice were perfused, and their spinal columns were postfixed with 4% PFA. The spinal cord segment under the laminectomy that had previously been imaged in vivo was dissected, paraffin-embedded, cut into 5-μm sections, stained with LFB and counterstained with Periodic Acid-Schiff (PAS) or immunostained with antibodies against fibrinogen (1:1,000), SMI-32 (1:1,000, Covance), Iba-1 (1:1,000, Wako), CD3 (1:1,000, Wako), or laminin (1:100, Sigma) as described [27] . Images were acquired with an Axioplan II epifluorescence microscope (Zeiss) equipped with dry Plan-Neofluar objectives (10 × 0.3 NA, 20 × 0.5 NA, or 40 × 0.75 NA). Quantification was performed on thresholded images using ImageJ. Correlated EM After in vivo imaging, mice were perfused and their spinal cord tissue was postfixed with 2.5% glutaraldehyde and 2% PFA in 0.1 M cacodylate buffer, pH 7.4, on ice. EM was performed with a JEM-1200EX electron microscope operated at 80 kV, according to standard procedures [58] . The negatives were digitized at 1800 dots per inch (dpi) with a Nikon CoolScan system. ROS detection Mice received daily i.p. injections of 25 mg kg −1 DHE (Invitrogen) for two consecutive days [59] . DHE was dissolved in 100% dimethyl sulfoxide (DMSO, Fisher) and further diluted in saline. BV2 microglial cells [27] were plated onto poly-d-lysine-coated cover glasses (Corning) in DMEM supplemented with 1% fetal FBS-HI, 100 U ml −1 penicillin and 100 mg ml −1 streptomycin. Cells were incubated with 5 μM H 2 O 2 probe PYME [60] for 30 min at 37 °C. After incubation, 1 μM fibrin d-dimer (HyTest) was added for 1 h, cells were washed, fixed with PFA and stained with IsoB4 (Sigma) as described [27] . Fibrin D -dimer is a fibrin degradation product that contains the binding sites of fibrinogen to CD11b/CD18 integrin, and it was used as a soluble alternative to fibrin. Real-time RT–PCR After 6 h of fibrin D -dimer (1 μM) treatment, total RNA was extracted from BV2 microglia with the RNeasy kit (QIAGEN). Reverse transcription and real-time PCR were performed as described [53] using the following primers: iNOS : forward, 5′-CAGCACAGGAAATGTTTCAGC-3′; reverse, 5′-TAGCCAGCGTACCGGATGA-3′; L7 : forward, 5′-GAAGCTCATCTATGAGAAGGC-3′; reverse, 5′-AAGACGAAGGAGCT GCAGAAC-3′. Results were analyzed with the StepOne Software (Applied Biosystems) using the comparative C T method [53] . Data were expressed as 2 −ΔΔC T for the experimental gene of interest, normalized against the mouse ribosomal protein L7 housekeeping gene and presented as fold change versus control. Statistical analyses Statistical significance was calculated with R (R foundation) or with GraphPad Prism (GraphPad), using unpaired t- test for normally distributed isolated pairs, Mann–Whitney test for non-normally distributed pairs, analysis of variance (one-way analysis of variance, Bonferroni post-test) for multiple comparisons, or two-way analysis of variance for examination of multiple observations on each independent variable. Linear regression correlation coefficients ( R 2 values) and P- values testing the null hypothesis that the overall slope is zero by F- test, were also calculated with GraphPad Prism. All analyses were performed in a given number of sections, clusters, or cells per spinal cord volume imaged in vivo , per mouse, and then calculated the mean±s.e.m. for the reported n numbers of animals per group. How to cite this article: Davalos D. et al . Fibrinogen-induced perivascular microglial clustering is required for the development of axonal damage in neuroinflammation. Nat. Commun. 3:1227 doi: 10.1038/ncomms2230 (2012).